TRAF6 ubiquitinates TGFβ type I receptor to promote its cleavage and nuclear translocation in cancer Transforming growth factor β (TGFβ) is a pluripotent cytokine promoting epithelial cell plasticity during morphogenesis and tumour progression. TGFβ binding to type II and type I serine/threonine kinase receptors (TβRII and TβRI) causes activation of different intracellular signaling pathways. TβRI is associated with the ubiquitin ligase tumor necrosis factor receptor (TNFR)-associated factor 6 (TRAF6). Here we show that TGFβ, via TRAF6, causes Lys63-linked polyubiquitination of TβRI, promoting cleavage of TβRI by TNF-alpha converting enzyme (TACE), in a PKCζ-dependent manner. The liberated intracellular domain (ICD) of TβRI associates with the transcriptional regulator p300 to activate genes involved in tumour cell invasiveness, such as Snail and MMP2. Moreover, TGFβ-induced invasion of cancer cells is TACE- and PKCζ- dependent and the TβRI ICD is localized in the nuclei of different kinds of tumour cells in tissue sections. Thus, our data reveal a specific role for TβRI in TGFβ mediated tumour invasion. Transforming growth factor β (TGFβ) is a cytokine which plays an important role during normal embryogenesis due to its multifunctional effects on cellular responses such as proliferation, differentiation, apoptosis and migration. In recent years TGFβ has become recognized as a potent regulator of cellular plasticity which is a central event during embryogenesis and tumour progression. TGFβ signals through its binding to the type II and type I serine/threonine kinase receptors (TβRII and TβRI, respectively), to cause their hetero-oligomerization which subsequently activates different intracellular signaling pathways. TβRI phosphorylates the latent transcription factors Smad2 and Smad3 in early endosomes, to induce complex formation with Smad4 and nuclear translocation to regulate target genes [1] , [2] , [3] , [4] . TβRI has been found to harbour a consensus binding site for the ubiquitin ligase tumor necrosis factor receptor (TNFR)-associated factor 6 (TRAF6); upon TGFβ binding TRAF6 activates the TGFβ activated kinase 1 (TAK1)—p38 mitogen activated protein (MAP) kinase pathway [5] , [6] . Interestingly, TNF-alpha converting enzyme (TACE) has recently been shown to cleave TβRI in its extracellular domain, which was demonstrated to cause a loss of TGFβ-induced inhibition of proliferation of cells [7] . Posttranslational modifications of proteins, such as monoubiquitination or Lys63-linked polyubiquitination, have emerged as an important mechanism to control the localization or function of the protein, whereas Lys48-linked polyubiquitination of proteins instead targets its substrate for proteasomal degradation [8] , [9] . TRAF6 is known to induce Lys63-linked polyubiquitination of its substrates, including TAK1 [5] . The underlying molecular mechanisms for how TGFβ can both act as a tumour suppressor and a promoter remain to be fully understood. To further address how TGFβ promotes tumour progression, we have investigated the possibility that TRAF6 regulates the subcellular localization of TβRI by Lys63-dependent polyubiquitination and whether this is related to the capability of TGFβ to facilitate tumour invasion. We report here that TGFβ uses TRAF6, PKCζ and TACE to promote the formation of an intracellular domain (ICD) of the TβRI that is translocated to the nucleus, where it promotes tumour invasion by induction of Snail and MMP2 . Nuclear accumulation of the intracellular domain of TβRI To investigate whether TβRI is proteolytically cleaved in human prostate cancer (PC-3U) cells, we ectopically expressed a C-terminally tagged constitutively active (ca) TβRI (HA-ALK5TD). Notably, in addition to the full length receptor, the HA antibody recognized a smaller fragment, corresponding to the estimated size of the intracellular part of TβRI ( Supplementary Fig. S1a ). Using immunofluorescence and confocal microscopy, we next investigated the subcellular localization of endogenous TβRI in PC-3U cells visualized by a antibodies raised against its intracellular, C-terminal part (V22) or its extracellular N-terminal part (H100; Fig. 1a ). An enhanced nuclear accumulation of TβRI, or its C-terminal fragment, was noticed in TGFβ-stimulated PC-3U cells, upon staining with the V22 antibody. In contrast, immunofluorescence staining revealed that the extracellular domain of the receptor, visualized by the H100-antibody was mainly localized in the cell membrane in PC-3U cells stimulated with TGFβ for 6 h ( Fig. 1a ). To ensure the specificity of the V22 antibody in immunofluorescence and immunoblotting, siRNA was used to knock-down endogenous TβRI expression in PC-3U cells ( Fig. 1a and Supplementary Fig. S1b ); qRT-PCR was also used to demonstrate a substantial decrease of TβRI mRNA expression ( Supplementary Fig. S1b ). The specificity of the V22 antibody used in our study was also verified by peptide blocking ( Supplementary Fig. S1c ). 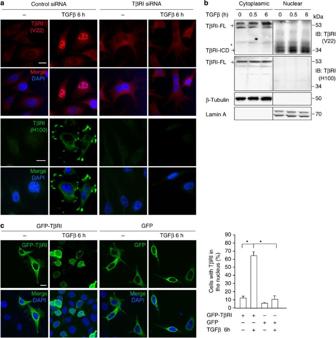Figure 1: TGFβ induces nuclear accumulation of TβRI intracellular domain (TβRI-ICD). (a,b) Knockdown of TβRI by siRNA was performed to demonstrate the specificity of the V22 and H100 antibodies, which recognize the intracellular and extracellular domain of TβRI, respectively, in immunofluorescence (a; DAPI was used to visualize cell nuclei, scale bar 20 μm). (b) Cell lysates of PC-3U cells treated or not with TGFβ, were fractionated into cytoplasmic and nuclear proteins and subjected to SDS–gel electrophoresis, followed by immunoblotting using V22 and H100 antibodies. β-tubulin and lamin A served as controls for the cytoplasmic and nuclear fractions, respectively. Molecular weight markers are indicated. (c) Representative confocal microscopy pictures of C-terminally pEGFP-N3-tagged wt TβRI (GFP- TβRI) and pEGFP-N3-vector (GFP) expressed in PC-3U cells treated with TGFβ for 6 h are shown (left panel) and quantified in right panel (mean±s.d.,n=3–5 independent experiments whereN=350 cells where counted in each group, *P<0.0002, ANOVA). Cell nuclei were stained with DAPI. Scale bar 20 μm. Figure 1: TGFβ induces nuclear accumulation of TβRI intracellular domain (TβRI-ICD). ( a , b ) Knockdown of TβRI by siRNA was performed to demonstrate the specificity of the V22 and H100 antibodies, which recognize the intracellular and extracellular domain of TβRI, respectively, in immunofluorescence ( a ; DAPI was used to visualize cell nuclei, scale bar 20 μm). ( b ) Cell lysates of PC-3U cells treated or not with TGFβ, were fractionated into cytoplasmic and nuclear proteins and subjected to SDS–gel electrophoresis, followed by immunoblotting using V22 and H100 antibodies. β-tubulin and lamin A served as controls for the cytoplasmic and nuclear fractions, respectively. Molecular weight markers are indicated. ( c ) Representative confocal microscopy pictures of C-terminally pEGFP-N3-tagged wt TβRI (GFP- TβRI) and pEGFP-N3-vector (GFP) expressed in PC-3U cells treated with TGFβ for 6 h are shown (left panel) and quantified in right panel (mean±s.d., n= 3–5 independent experiments where N =350 cells where counted in each group, * P <0.0002, ANOVA). Cell nuclei were stained with DAPI. Scale bar 20 μm. Full size image To further validate the observation that TβRI, or its intracellular domain (ICD), is translocated to the nucleus in a TGFβ-dependent manner, we performed a nuclear fractionation assay of cell lysates from TGFβ-treated PC-3U cells. Immunoblotting of nuclear extracts by the V22 antibody revealed a TβRI fragment of approximally 34 kDa, which was not recognized by the H100 antibody raised against the N-terminal part of TβRI ( Fig. 1b ). In contrast, full-length TβRI was observed in the cytoplasmic fraction, both by the V22 and H100 antibodies ( Fig. 1b ). While a pronounced increase of nuclear TβRI was detected by immunofluorescence only after TGFβ stimulation ( Fig. 1a ), nuclear TβRI was detected by immunoblotting also in the absence of TGFβ stimulation ( Fig. 1b ). This discrepancy is probably due to the fact that sensitivity for detection of nuclear TβRI is higher with the nuclear fractionation assay. To further investigate the TGFβ-dependency of nuclear accumulation of TβRI, we expressed a fusion protein in which GFP was linked to the C-terminal part of TβRI in PC-3U cells. The GFP-tagged TβRI entered the nucleus of PC-3U cells after stimulation with TGFβ for 6 h, while GFP expressed from a vector containing GFP alone did not ( Fig. 1c ). We also investigated the nuclear localization of ectopically expressed C-terminally HA-tagged ca TβRI in PC-3U cells and observed a TGFβ-induced accumulation of the HA-tagged ca TβRI-ICD ( Supplementary Fig. S1d ). This observation is consistent with the nuclear accumulation of endogenous TβRI-ICD as shown in Figure 1a,b . In further support of the notion that the N-terminal part of the TβRI did not enter the nucleus, a HA-tagged TβRI with the tag localized N-terminally between amino acid residues 27 and 28 [4] , was found not to enter the nucleus in PC-3U cells with or without treatment with TGFβ ( Supplementary Fig. S1e ). Moreover, no TGFβ-induced increase of the TβRI-ICD for N-terminal HA-tagged TβRI was observed ( Supplementary Fig. S1f ). Together, these results suggest that the ICD of TβRI enters into the nucleus in PC-3U cells in response to TGFβ stimulation. Nuclear accumulation of TβRI is dependent on TRAF6 We have recently identified a consensus binding site for TRAF6 in TβRI [5] . Ligand-induced oligomerization of the TGFβ receptor complex results in receptor kinase-independent activation of the enzymatic activity of TRAF6. This in turn causes Lys63-polyubiquitin-dependent activation of TGFβ-activated kinase-1 (TAK1), causing activation of p38 MAPK in PC-3U cells. In contrast, activation of the canonical Smad pathway does not require TRAF6 [5] . To examine whether TRAF6 is important for the cleavage and nuclear accumulation of TβRI, we expressed C-terminally HA-tagged wild-type (wt) caTβRI (HA-TβRI) or the HA-tagged caE161A (HA-E161A) receptor mutant which is unable to bind TRAF6, but still causes activation of the canonical Smad signalling pathway [5] . 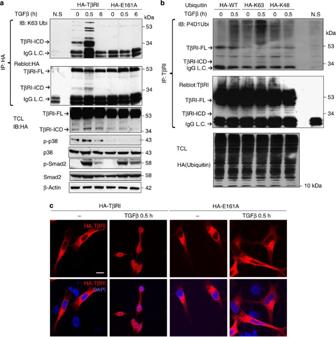Figure 2: TRAF6 promotes Lys63-dependent polyubiquitination of wt TβRI but not of the E161A mutant TβRI. (a) PC-3U cells transiently transfected with C-terminally HA-tagged wt TβRI, or E161A mutant TβRI deficient in association with TRAF6, were treated or not with TGFβ, whereafter ubiquitination of TβRI was examined by anin vivoubiquitination assay. Complexes immunoprecipitated (IP) with anti-HA antibodies were immunoblotted (IB) with Lys63 (K63)-linked polyubiquitin-specific antibody. A light-chain specific secondary antiserum was used to avoid cross-reaction with IgG heavy chain. Molecular weight markers are indicated. Another part of the corresponding total cell lysates (TCL) was subjected to immunoblotting for HA to detect the TβRI-ICD fragment, and activation of p38 and Smad2, by phospho-specific antisera. The filters were then reprobed with total p38 or Smad2, to verify specificity of phospho-specific antisera and actin served as internal control for equal loading of proteins. (b)In vivoubiquitination assays performed in PC-3U cells transiently transfected with HA-tagged wt, K63- and K48-only ubiquitin. Cell lysates were immunoprecipitated with V22 antibody against TβRI, and K63-dependent polyubiquitination was visualized by immunoblotting with P4D1-antiserum. A light-chain specific secondary antiserum was used to avoid cross-reaction with IgG heavy chain. The TCL-filter was subjected to immunoblotting with an HA-antibody to verify equal expression levels of ubiquitin. (c) PC-3U cells ectopically expressing C-terminally HA-tagged wt TβRI or the corresponding E161A mutant were stimulated with TGFβ for 0.5 h and thereafter stained with an HA antibody. Staining with DAPI was used to visualize cell nuclei. Scale bar 20 μm. As shown in Figure 2a , stimulation of cells with TGFβ resulted in Lys63-linked polyubiquitination of wt TβRI, but not of the E161A mutant TβRI. Cleavage of the wt TβRI, as observed by immunoblotting of total cell lysate with HA antiserum was found to associate with its Lys63-linked polyubiquitination ( Fig. 2a ). Moreover, the E161A mutant TβRI failed to activate the p38 MAPK pathway while it was still able to activate Smad2, consistent with our previous report [5] ( Fig. 2a ). In addition, knock-down of endogenous TRAF6 in PC-3U cells by siRNA, also resulted in loss of Lys63-linked polyubiquitination of TβRI, as well as loss of the formation of the TβRI ICD in response to stimulation with TGFβ ( Supplementary Fig. S2a,b ). By using either Lys63 or Lys48 polyubiquitin-specific antibodies, we found that wt TβRI was Lys63-polyubiquitinated after 30 min of TGFβ stimulation, while no obvious sign of TGFβ-induced Lys48-polyubiqutination of TβRI, was observed in this cell line during this time course ( Fig. 2a and Supplementary Fig. S2a,c ). Figure 2: TRAF6 promotes Lys63-dependent polyubiquitination of wt TβRI but not of the E161A mutant TβRI. ( a ) PC-3U cells transiently transfected with C-terminally HA-tagged wt TβRI, or E161A mutant TβRI deficient in association with TRAF6, were treated or not with TGFβ, whereafter ubiquitination of TβRI was examined by an in vivo ubiquitination assay. Complexes immunoprecipitated (IP) with anti-HA antibodies were immunoblotted (IB) with Lys63 (K63)-linked polyubiquitin-specific antibody. A light-chain specific secondary antiserum was used to avoid cross-reaction with IgG heavy chain. Molecular weight markers are indicated. Another part of the corresponding total cell lysates (TCL) was subjected to immunoblotting for HA to detect the TβRI-ICD fragment, and activation of p38 and Smad2, by phospho-specific antisera. The filters were then reprobed with total p38 or Smad2, to verify specificity of phospho-specific antisera and actin served as internal control for equal loading of proteins. ( b ) In vivo ubiquitination assays performed in PC-3U cells transiently transfected with HA-tagged wt, K63- and K48-only ubiquitin. Cell lysates were immunoprecipitated with V22 antibody against TβRI, and K63-dependent polyubiquitination was visualized by immunoblotting with P4D1-antiserum. A light-chain specific secondary antiserum was used to avoid cross-reaction with IgG heavy chain. The TCL-filter was subjected to immunoblotting with an HA-antibody to verify equal expression levels of ubiquitin. ( c ) PC-3U cells ectopically expressing C-terminally HA-tagged wt TβRI or the corresponding E161A mutant were stimulated with TGFβ for 0.5 h and thereafter stained with an HA antibody. Staining with DAPI was used to visualize cell nuclei. Scale bar 20 μm. Full size image The pattern of polyubiquitination of TβRI was further examined using HA-tagged wt or mutant ubiquitin overexpressed in PC-3U cells. TGFβ stimulation induced polyubiquitination of TβRI in PC-3U cells transiently transfected with a ubiquitin mutant in which all lysine residues where mutated except Lys63, while reduced ubiquitination was seen when a similar mutant retaining only Lys48 was expressed ( Fig. 2b ). In addition, TRAF6 was shown to induce the polyubiquitination of TβRI in an in vitro ubiquitination assay, providing firm evidence that TβRI is a substrate for TRAF6 ( Supplementary Fig. S3 ). TGFβ-induced nuclear accumulation of ectopically expressed C-terminal HA-tagged caTβRI in PC-3U cells occurred more efficiently for the wt TβRI than for the E161A mutant HA-TβRI, as analyzed by immunofluorescence ( Fig. 2c ). On the basis of these data, we conclude that TRAF6 causes Lys63-dependent polyubiquitination of TβRI in a TGFβ-dependent manner which correlates with generation of an intracellular fragment of TβRI and its nuclear accumulation. TβRI is cleaved by TACE The metalloproteases TNF-alpha converting enzyme (TACE)/ADAM17 and ADAM10, when activated, cleave certain receptors and adhesion proteins, just outside the cell membrane. TACE has recently been shown to cleave TβRI in an ERK MAP-kinase dependent manner, leading to desensitization of TGFβ signaling [7] . TACE is often overexpressed in tumours and is activated by PKC [10] . To further characterize the molecular mechanisms behind the cleavage and nuclear translocation of TβRI, we examined the possible involvement of the metalloproteinase TACE/ADAM17. Treatment of human PC-3U cells with TPA to activate PKC [10] led to nuclear accumulation of endogenous TβRI or its ICD, as shown by immunofluorescence ( Fig. 3a ). Moreover, when PC-3U cells expressing the C-terminally tagged HA-caTβRI were treated with TGFβ or TPA, the ICD accumulated in the nuclear fraction ( Fig. 3b ). Pretreatment of cells with TAPI-2, an inhibitor of TACE, led to a decreased nuclear entrance of the ICD of endogenous TβRI in response to TGFβ stimulation ( Fig. 3c,d ). As TACE was shown recently to associate with the ectopically expressed TβRI in cells expressing HER2 [11] , we investigated by co-immunofluorescence if endogenous TβRI associated with TACE in PC-3U cells. A TGFβ-induced colocalization of TβRI and TACE was observed ( Fig. 3e ). From these data, we conclude that activation of TACE, either by TPA-treatment of cells or stimulation with TGFβ, leads to accumulation of the TβRI ICD in the nucleus. 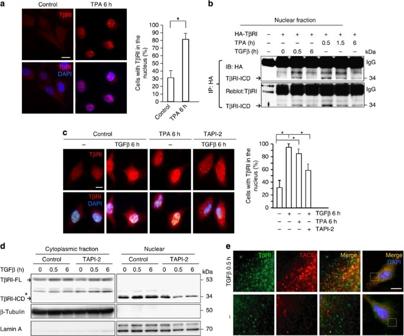Figure 3: TACE regulates nuclear accumulation of TβRI ICD. (a) PC-3U cells were treated with TPA for 6 h. Endogenous TβRI is shown by immunofluorescence using the V22 antibody. Quantification of the number of cells showing endogenous TβRI in the nucleus is shown on the right side of the panel (mean±s.d.,n=3 independent experiment, whereN=200–300 cells where counted in each group, *P<0.0001, ANOVA). Scale bar 20 μm. (b) Nuclear proteins from PC-3U cells transiently transfected with C-terminally HA-tagged TβRI were treated as indicated, then samples were subjected to immunoprecipitation with an HA antibody. The TβRI-ICD was visualized by immunoblotting with an HA antibody and the membrane was thereafter stripped and reblotted with VPN antiserum against the intracellular part of the receptor. (c) PC-3U cells were treated with either TGFβ or TPA alone for 6 h or with both TGFβ and TAPI-2 for 6 h. Endogenous TβRI is shown by immunofluorescence using the V22 antibody. Quantification of the number of cells showing endogenous TβRI in the nucleus is shown on the right side of the panel (mean±s.d,n=3 independent experiments, whereN=200–300 cells where counted from each group, *P<0.0001, ANOVA). Scale bar 20 μm. (d) Cell lysates of PC-3U cells treated with TGFβ in the presence or absence of TAPI-2 as indicated, were fractionated into cytoplasmic and nuclear proteins and subjected to SDS-gel electrophoresis, followed by immunoblotting using V22 antibody, which recognizes both the TβRI full length (TβRI-FL) and intracellular domain of TβRI (TβRI-ICD). β-tubulin and lamin A served as controls for the cytoplasmic and nuclear fractions, respectively. Molecular weight markers are indicated. *indicates a background band. (e) PC-3U cells were with treated or not with TGFβ for 0.5 h. Endogenous TACE and TβRI are shown by co-immunofluorescence using TACE (TRITC) and V22 (FITC) antisera. Their colocalization is demonstrated by the yellow colour as shown in merge. The pictures are enlargements of the picture to the right (white box). Scale bar 20 μm. Stainings with DAPI was used to visualize cell nuclei in (a,cande). Figure 3: TACE regulates nuclear accumulation of TβRI ICD. ( a ) PC-3U cells were treated with TPA for 6 h. Endogenous TβRI is shown by immunofluorescence using the V22 antibody. Quantification of the number of cells showing endogenous TβRI in the nucleus is shown on the right side of the panel (mean±s.d., n =3 independent experiment, where N =200–300 cells where counted in each group, * P <0.0001, ANOVA). Scale bar 20 μm. ( b ) Nuclear proteins from PC-3U cells transiently transfected with C-terminally HA-tagged TβRI were treated as indicated, then samples were subjected to immunoprecipitation with an HA antibody. The TβRI-ICD was visualized by immunoblotting with an HA antibody and the membrane was thereafter stripped and reblotted with VPN antiserum against the intracellular part of the receptor. ( c ) PC-3U cells were treated with either TGFβ or TPA alone for 6 h or with both TGFβ and TAPI-2 for 6 h. Endogenous TβRI is shown by immunofluorescence using the V22 antibody. Quantification of the number of cells showing endogenous TβRI in the nucleus is shown on the right side of the panel (mean±s.d, n =3 independent experiments, where N =200–300 cells where counted from each group, * P <0.0001, ANOVA). Scale bar 20 μm. ( d ) Cell lysates of PC-3U cells treated with TGFβ in the presence or absence of TAPI-2 as indicated, were fractionated into cytoplasmic and nuclear proteins and subjected to SDS-gel electrophoresis, followed by immunoblotting using V22 antibody, which recognizes both the TβRI full length (TβRI-FL) and intracellular domain of TβRI (TβRI-ICD). β-tubulin and lamin A served as controls for the cytoplasmic and nuclear fractions, respectively. Molecular weight markers are indicated. *indicates a background band. ( e ) PC-3U cells were with treated or not with TGFβ for 0.5 h. Endogenous TACE and TβRI are shown by co-immunofluorescence using TACE (TRITC) and V22 (FITC) antisera. Their colocalization is demonstrated by the yellow colour as shown in merge. The pictures are enlargements of the picture to the right (white box). Scale bar 20 μm. Stainings with DAPI was used to visualize cell nuclei in ( a , c and e ). Full size image Determination of the TACE cleavage site in TβRI Previous studies have shown that TACE has a strong preference for cleavage at Ala-Val sequences [12] or Gly-Leu sequences [13] . TβRI contains two Gly-Leu sequences, located at position Gly52 and Gly120. To investigate the possibility that TACE cleaves TβRI at Gly120, which is located close to the transmembrane domain, we mutated Gly 120 to Ile (G120I) in TβRI. The G120I mutant TβRI did not undergo cleavage in response to TGFβ stimulation ( Fig. 4a ), suggesting that TACE cleaves TβRI at the Gly-Leu bond at position 120–121. The kinase activity of the G120I mutant was intact as judged by its ability to phosphorylate Smad2, when compared with wt TβRI. Moreover, the G120I mutant TβRI did not accumulate in the nucleus in response to TGFβ stimulation ( Fig. 4b ). 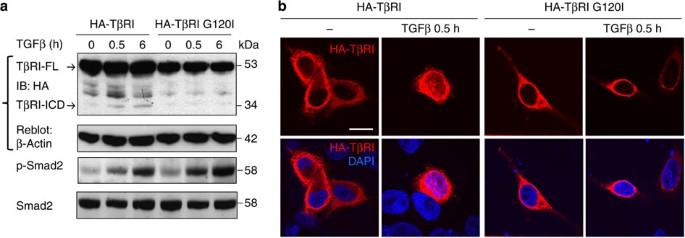Figure 4: Identification of the TGFβ-induced cleavage site for TACE in the extracellular domain of TβRI. (a) Total cell lysates derived from PC-3U cells transiently transfected with C-terminally HA-tagged wt TβRI or the corresponding G120I mutant were stimulated with TGFβ as indicated, was subjected to immunoblotting for HA to detect the TβRI-ICD fragment. The filter was reprobed with β-actin antibodies to show equal loading of proteins in all lanes, and activation of Smad2, by a phospho-specific antiserum (p-Smad2). The p-Smad2 filter was reblotted with total Smad2. (b) Representative confocal microscopy pictures of PC-3U cells ectopically expressing C-terminally HA-tagged wt TβRI or the corresponding G120I mutant were stimulated with TGFβ for 0.5 h and thereafter stained with HA antibody. Staining with DAPI was used to visualize cell nuclei. Scale bar 20 μm. Figure 4: Identification of the TGFβ-induced cleavage site for TACE in the extracellular domain of TβRI. ( a ) Total cell lysates derived from PC-3U cells transiently transfected with C-terminally HA-tagged wt TβRI or the corresponding G120I mutant were stimulated with TGFβ as indicated, was subjected to immunoblotting for HA to detect the TβRI-ICD fragment. The filter was reprobed with β-actin antibodies to show equal loading of proteins in all lanes, and activation of Smad2, by a phospho-specific antiserum (p-Smad2). The p-Smad2 filter was reblotted with total Smad2. ( b ) Representative confocal microscopy pictures of PC-3U cells ectopically expressing C-terminally HA-tagged wt TβRI or the corresponding G120I mutant were stimulated with TGFβ for 0.5 h and thereafter stained with HA antibody. Staining with DAPI was used to visualize cell nuclei. Scale bar 20 μm. Full size image PKCζ is needed for TACE-induced cleavage of TβRI We next investigated whether PKCζ, which is the only member in the PKC-family known to form a multiprotein-complex with TRAF6 [14] , is involved in cleavage of TβRI and nuclear translocation of the ICD. Inhibition of PKCζ, by PKCζ pseudosubstrate, completely prevented nuclear accumulation of the TβRI ICD in a dose-dependent manner ( Fig. 5a and Supplementary Fig. S4a ). It is well accepted that the classical members of the PKC family are activated by TPA, while atypic PKC isoforms like PKCζ are thought not to be activated by TPA [15] , [16] . However, we found that PKCζ is activated as a result of stimulation of cells by TGFβ, as well as by TPA ( Fig. 5b ). TGFβ stimulation did not lead to activation of PKCζ in TRAF6 −/− MEFs ( Fig. 5c ), supporting the notion that TRAF6 is important for TGFβ-induced activation of PKCζ. Using a nuclear fractionation assay, we noticed a significant loss of TGFβ-induced nuclear accumulation of TβRI ICD after siRNA-mediated silencing of PKCζ ( Fig. 5d ). In addition, ectopic expression of wt PKCζ promoted expression and cleavage of caTβRI or kinase dead (KD) TβRI mutant ( Fig. 5e ). Treatment of PC-3U cells with the PKCζ inhibitor decreased the formation of the ICD of C-terminally HA-tagged ca TβRI in TGFβ-treated cells as well as in a dose-dependent manner ( Supplementary Fig. S4b,c ), while treatment with the TβRI kinase inhibitor SB505124 had no major effect ( Fig. 5f ). 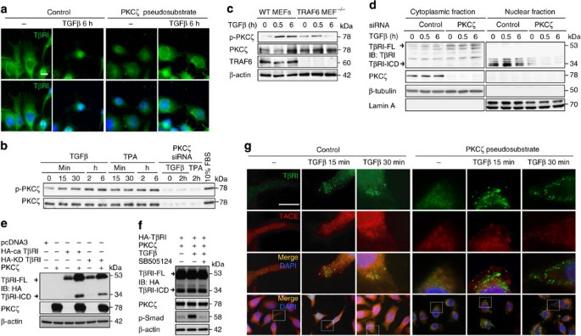Figure 5: PKCζ promotes nuclear accumulation of TβRI. (a) Immunofluorescence of endogenous TβRI visualized with the V22 antibody in PC-3U cells treated with TGFβ with or without PKCζ pseudosubstrate to inhibit PKCζ. Scale bar 20 μm. (b) Cell lysates from PC-3U cells treated with TGFβ or TPA were subjected to immunoblotting with pPKCζ antibody. Total cell lysates from cells transiently transfected with PKCζ siRNA served as negative control and cells treated with 10% FBS as positive control. The filter was reprobed with PKCζ antiserum to show equal loading of proteins in all lanes. (c) Cell lysates from wt and TRAF6−/−MEFs was subjected to immunoblotting for p-PKCζ,/PKCζ, TRAF6 and β-actin antibodies to show activation of PKCζ, knock down of TRAF6, and equal loading of proteins in all lanes, respectively. (d) PC-3U cells, in which endogenous PKCζ was silenced by its siRNA or not, and then treated with TGFβ, were subjected to cell fractionation followed by SDS–gel electrophoresis and immunoblotting to investigate the subcellular localization of endogenous TβRI. Lamin A and β-tubulin served as controls for the nuclear and cytoplasmic fractions, respectively. (e) Cell lysates from PC-3U cells transiently transfected and treated as indicated, in the presence or absence of wt PKCζ, subjected to immunoblotting to visualize TβRI-FL and TβRI-ICD. Immunoblotting of cell lysates for PKCζ and β-actin served as controls for the experiment. (f) Cell lysates from PC-3U cells transiently transfected with C-terminally HA-tagged wt TβRI and wt PKCζ, and treated with TGFβ in the presence and absence of TβRI inhibitor (SB505124) , subjected to immunoblotting for HA to visualize TβRI-FL and TβRI-ICD. Immunoblotting of cell lysates for PKCζ, p-Smad2 and β-actin served as controls for the experiment. (g) PC-3U cells were treated with TGFβ, with or without the PKCζ pseudosubstrate. Endogenous TACE and TβRI were visualized by immunofluorescence using TACE (TRITC) and V22 (FITC) antisera. Their colocalization is demonstrated by the yellow colour as shown in merge. Scale bar 20 μm. Stainings with DAPI was used to visualize cell nuclei ina,g. Figure 5: PKCζ promotes nuclear accumulation of TβRI. ( a ) Immunofluorescence of endogenous TβRI visualized with the V22 antibody in PC-3U cells treated with TGFβ with or without PKCζ pseudosubstrate to inhibit PKCζ. Scale bar 20 μm. ( b ) Cell lysates from PC-3U cells treated with TGFβ or TPA were subjected to immunoblotting with pPKCζ antibody. Total cell lysates from cells transiently transfected with PKCζ siRNA served as negative control and cells treated with 10% FBS as positive control. The filter was reprobed with PKCζ antiserum to show equal loading of proteins in all lanes. ( c ) Cell lysates from wt and TRAF6 −/− MEFs was subjected to immunoblotting for p-PKCζ,/PKCζ, TRAF6 and β-actin antibodies to show activation of PKCζ, knock down of TRAF6, and equal loading of proteins in all lanes, respectively. ( d ) PC-3U cells, in which endogenous PKCζ was silenced by its siRNA or not, and then treated with TGFβ, were subjected to cell fractionation followed by SDS–gel electrophoresis and immunoblotting to investigate the subcellular localization of endogenous TβRI. Lamin A and β-tubulin served as controls for the nuclear and cytoplasmic fractions, respectively. ( e ) Cell lysates from PC-3U cells transiently transfected and treated as indicated, in the presence or absence of wt PKCζ, subjected to immunoblotting to visualize TβRI-FL and TβRI-ICD. Immunoblotting of cell lysates for PKCζ and β-actin served as controls for the experiment. ( f ) Cell lysates from PC-3U cells transiently transfected with C-terminally HA-tagged wt TβRI and wt PKCζ, and treated with TGFβ in the presence and absence of TβRI inhibitor (SB505124) , subjected to immunoblotting for HA to visualize TβRI-FL and TβRI-ICD. Immunoblotting of cell lysates for PKCζ, p-Smad2 and β-actin served as controls for the experiment. ( g ) PC-3U cells were treated with TGFβ, with or without the PKCζ pseudosubstrate. Endogenous TACE and TβRI were visualized by immunofluorescence using TACE (TRITC) and V22 (FITC) antisera. Their colocalization is demonstrated by the yellow colour as shown in merge. Scale bar 20 μm. Stainings with DAPI was used to visualize cell nuclei in a , g . Full size image Using immunofluorescence stainings, we observed TGFβ-induced co-localization of endogenous TβRI and TACE. Adding the PKCζ pseudosubstrate to cells prevented the co-localization ( Fig. 5g ), suggesting that PKCζ activity is needed for a proper localization of TβRI to a subcellular compartment where it can be cleaved by TACE. In conclusion, TGFβ causes activation of PKCζ in a TRAF6-dependent manner, which is important for the proteolytic cleavage of the TβRI by TACE, leading to nuclear accumulation of TβRI ICD. TβRI ICD regulates transcription The observation that the ICD of TβRI enters the nucleus in TGFβ-treated PC-3U cells, suggests that it might participitate in gene regulation. To search for a link between the nuclear TβRI ICD and gene transcription, we investigated if TβRI ICD associates with the well-known transcriptional regulator p300. TGFβ treatment of PC-3U cells led to a co-localization of TβRI and p300 in nuclear specles ( Fig. 6a ), which we identified by co-immunofluorescence as promyelocytic leukemia protein (PML) nuclear bodies [17] ( Fig. 6b ). Treatment of cells with the PKCζ pseudosubstrate prevented the co-localization of TβRI with PML nuclear bodies ( Fig. 6b ). By co-immunoprecipitation experiments, the acetyltransferase p300 was found to associate with TβRI ICD in vivo ( Fig. 6c,d ) and we used an acetyl-lysine antibody to verify that TβRI ICD is acetylated ( Fig. 6e ). In contrast, in cells expressing the E161A mutant TβRI, less ICD was associated with endogenous p300 and less acetylated ICD was detected ( Fig. 6d,e ). We observed that the level of p300 was lower in cells transfected with the E161A mutant TβRI unable to bind TRAF6, compared to wt TβRI ( Fig. 6d ). Using qRT-PCR, a TGFβ-induced increase of p300 mRNA expression was observed in cells transiently transfected with wt TβRI, but not in cells transfected with E161A mutant TβRI ( Fig. 6f ). This suggests that TGFβ induces p300 in a TRAF6-dependent manner. 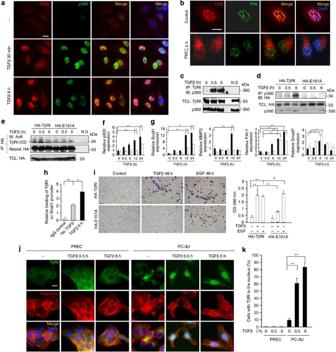Figure 6: TβRI promotes expression of Snail and invasion of prostate cancer cells in a TGFβ-dependent manner. (a) PC-3U cells were treated with or without TGFβ. Endogenous TβRI and p300 are visualized by immunofluorescence using V22 (TRITC) and p300 (FITC) antibodies. Note the TGFβ-induced nuclear accumulation of endogenous TβRI and colocalization with p300 (shown in merge; yellow). (b) PC-3U cells were treated as indicated. Endogenous TβRI and PML are shown by immunofluorescence using V22 (TRITC) and PML (FITC) antisera. (c) TGFβ induces association between endogenous TβRI and p300. Cell lysates from PC-3U cells treated with TGFβ were immunoprecipitated with the V22 antibody against TβRI and subjected to immunoblotting with p300 antibody. (d) Cell lysates from PC-3U cells transiently transfected and treated as indicated, were immunoprecipitated with an antibody against p300 and subjected to immunoblotting with HA antibody. (e) Cell lysates from PC-3U cells, transiently transfected and treated as indicated, were immunoprecipitated with an antibody against HA and subjected to immunoblotting with acetyl-Lys (AcK) antibody. (f,g) qRT-PCR analysis for expression ofp300,Snail-1,MMP2,PAI1andSmad7was performed on mRNA extracted from PC-3U cells transiently transfected with wt HA-TβRI (filled bars) or the E161A mutant (open bars) and treated as indicated. (h) Chromatin immunoprecipitation assay for theSnailpromoter using V22 antibody against the endogenous TβRI in PC-3U cells treated or not with TGFβ. (i) Invasion assay for PC-3U cells, transiently transfected and treated as indicated. Cells were visualized by staining with crystal violet cell stain solution. Right panel presents mean values for optical density (OD) of invasive cells. (j) Immunofluorescence stainings of cytoskeletal reorganization of actin and subcellular localization of TβRI in TGFβ-treated primary prostate epithelial cells (PREC) and PC-3U cells for comparison. (k) Quantification of the number of cells in (j) showing endogenous TβRI in the nucleus, whereN=200 cells were counted in each group. (a,b,j) Staining with DAPI was used to visualize cell nuclei. Scale bar 20 μm. Data in (f,g,h,i,k) are representative of three independent experiments (mean and s.d). *P<0.05 and **P<0.005 (ANOVA except for relative Smad7 expression, where Studentst-test were used). Figure 6: TβRI promotes expression of Snail and invasion of prostate cancer cells in a TGFβ-dependent manner. ( a ) PC-3U cells were treated with or without TGFβ. Endogenous TβRI and p300 are visualized by immunofluorescence using V22 (TRITC) and p300 (FITC) antibodies. Note the TGFβ-induced nuclear accumulation of endogenous TβRI and colocalization with p300 (shown in merge; yellow). ( b ) PC-3U cells were treated as indicated. Endogenous TβRI and PML are shown by immunofluorescence using V22 (TRITC) and PML (FITC) antisera. ( c ) TGFβ induces association between endogenous TβRI and p300. Cell lysates from PC-3U cells treated with TGFβ were immunoprecipitated with the V22 antibody against TβRI and subjected to immunoblotting with p300 antibody. ( d ) Cell lysates from PC-3U cells transiently transfected and treated as indicated, were immunoprecipitated with an antibody against p300 and subjected to immunoblotting with HA antibody. ( e ) Cell lysates from PC-3U cells, transiently transfected and treated as indicated, were immunoprecipitated with an antibody against HA and subjected to immunoblotting with acetyl-Lys (AcK) antibody. ( f , g ) qRT-PCR analysis for expression of p300 , Snail-1 , MMP2 , PAI1 and Smad7 was performed on mRNA extracted from PC-3U cells transiently transfected with wt HA-TβRI (filled bars) or the E161A mutant (open bars) and treated as indicated. ( h ) Chromatin immunoprecipitation assay for the Snail promoter using V22 antibody against the endogenous TβRI in PC-3U cells treated or not with TGFβ. ( i ) Invasion assay for PC-3U cells, transiently transfected and treated as indicated. Cells were visualized by staining with crystal violet cell stain solution. Right panel presents mean values for optical density (OD) of invasive cells. ( j ) Immunofluorescence stainings of cytoskeletal reorganization of actin and subcellular localization of TβRI in TGFβ-treated primary prostate epithelial cells (PREC) and PC-3U cells for comparison. ( k ) Quantification of the number of cells in ( j ) showing endogenous TβRI in the nucleus, where N =200 cells were counted in each group. ( a , b , j ) Staining with DAPI was used to visualize cell nuclei. Scale bar 20 μm. Data in ( f , g , h , i , k ) are representative of three independent experiments (mean and s.d). * P <0.05 and ** P <0.005 (ANOVA except for relative Smad7 expression, where Students t -test were used). Full size image Next, we used qRT-PCR to analyze the effect of TβRI ICD on known TGFβ target genes. Snail and MMP2 mRNA expressions were induced by wt TβRI but much less by the E161A mutant TβRI, whereas PAI1 and Smad7 were induced by both wt and E161A mutant TβRI ( Fig. 6g ). A chromatin immunoprecipitation (ChIP) assay revealed binding of TβRI or TβRI ICD to the endogenous Snail promoter in a TGFβ-dependent manner in PC-3U cells ( Fig. 6h ). Since expression of Snail and MMP2 genes is linked to tumour invasiveness [18] , we examined PC-3U cells expressing wt or E161A mutant TβRI using an invasion assay. Interestingly, we observed that TGFβ-induced invasion occurred in PC-3U cells only when wt TβRI was expressed, whereas epidermal growth factor (EGF) stimulated invasion both in cells expressing wt or mutant TβRI ( Fig. 6i , right panel shows optical density (OD) mean values of stained invasive tumour cells). Similar results were observed when the experiment was repeated using the human prostate cancer cell line LNCaP; TGFβ treatment of LNCaP cells expressing wt TβRI, but not the E161A mutant TβRI, promoted their invasion ( Supplementary Fig. S5a,b ). Thus, our data propose that the TβRI ICD associates with p300 in nuclear PML bodies in a PKCζ-dependent manner, and is acetylated by p300. Moreover, Snail and MMP2 are induced by TβRI ICD, correlating with an increased invasiveness of cells. Nuclear TβRI ICD is observed in malignant prostate cells We observed that the nuclear entrance of TβRI was associated with invasiveness of prostate cancer cells; therefore, we used immunofluorescence and confocal microscopy to investigate the subcellular localization of endogenous TβRI, in primary human prostate epithelial cells (PrEC) cells and PC-3U cells, visualized by the V22 antibody raised against its C-terminal part ( Fig. 6j,k ). Intriguingly, accumulation of TβRI or its ICD in the nucleus took place in malignant PC-3U cells, but not in normal PrEC cells, where TβRI was retained in cell-cell contacts, also after treatment with TGFβ. Nuclear TβRI ICD is linked to TGFβ-induced cancer invasion To explore the generality of the TGFβ-induced pathway identified in this report, we extended our investigation to the human breast carcinoma cell line MDA-MB-231 and the human lung carcinoma cell line A549. By using confocal imaging, we found that TGFβ treatment of MDA-MB-231 also promotes accumulation of endogenous ICD of TβRI in the nucleus, in a TACE- and PKCζ- dependent manner, which was found to be associated with the TGFβ-induced invasiveness of the cells ( Fig. 7a,b ). We observed a similar association between TGFβ-induced nuclear accumulation of TβRI ICD and TGFβ-induced invasiveness in the A549 cell line, which also in these cancer cells were regulated by TACE and PKCζ ( Fig. 7c,d ). From these data we conclude that TGFβ-induced invasion of human breast and lung cancer cells correlates with nuclear accumulation of TβRI in a TACE- and PKCζ-dependent manner. 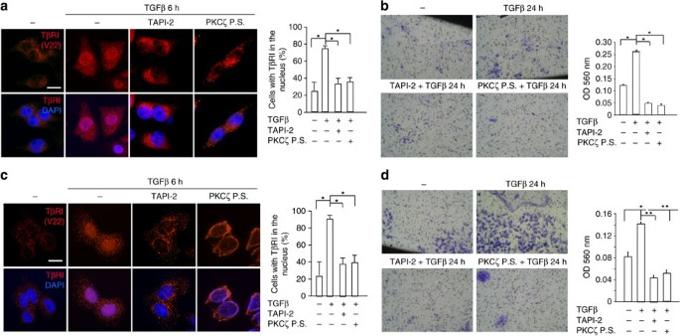Figure 7: TβRI nuclear localization in human breast and lung carcinoma cells is associated with tumour invasion. (a) Human breast carcinoma (MDA-MB-231) cells were starved and treated with TGFβ in the presence or absence of the PKCζ pseudosubstrate (P.S.) or TAPI-2, as indicated. Endogenous C-terminal TβRI was visualized by immunofluorescence using the V22 antibody (TRITC). Quantification of the number of cells showing endogenous TβRI in the nucleus is shown on the right side of the panel (mean±s.d.,n=3 independent experiment, whereN=200–300 cells where counted in each group, *P<0.001, ANOVA). Scale bar 20 μm. (b) Invasion assay for MDA-MB-231 treated with TGFβ in the absence or presence of TAPI-2 and PKCζ P.S. Cells were visualized by staining with crystal violet cell stain solution. Right panel presents mean values for optical density (OD) of invasive cells. Error bars represents s.d. (n=3 independent experiments, *P<0.05; Studentst-test). (c) Human lung carcinoma (A549) cell were starved and treated with TGFβ in the presence or absence of the PKCζ P.S or TAPI-2, as indicated. Endogenous C-terminal TβRI was visualized by immunofluorescence using the V22 antibody (TRITC). Quantification of the number of cells showing endogenous TβRI in the nucleus is shown on the right side of the panel (mean±s.d.,n=3 independent experiment, where N=200-300 cells where counted in each group, *P<0.0003, ANOVA). Scale bar 20 μm. (d) Invasion assay for A549 cells treated with TGFβ in the absence or presence of TAPI-2 and PKCζ P.S. Cells were visualized by staining with crystal violet cell stain solution. Right panel presents mean values for OD of invasive cells. Error bars represents mean±s.d. (n=3 independent experiments; *P<0.05, **P<0.002, ANOVA). Figure 7: TβRI nuclear localization in human breast and lung carcinoma cells is associated with tumour invasion. ( a ) Human breast carcinoma (MDA-MB-231) cells were starved and treated with TGFβ in the presence or absence of the PKCζ pseudosubstrate (P.S.) or TAPI-2, as indicated. Endogenous C-terminal TβRI was visualized by immunofluorescence using the V22 antibody (TRITC). Quantification of the number of cells showing endogenous TβRI in the nucleus is shown on the right side of the panel (mean±s.d., n =3 independent experiment, where N =200–300 cells where counted in each group, * P <0.001, ANOVA). Scale bar 20 μm. ( b ) Invasion assay for MDA-MB-231 treated with TGFβ in the absence or presence of TAPI-2 and PKCζ P.S. Cells were visualized by staining with crystal violet cell stain solution. Right panel presents mean values for optical density (OD) of invasive cells. Error bars represents s.d. ( n =3 independent experiments, * P <0.05; Students t -test). ( c ) Human lung carcinoma (A549) cell were starved and treated with TGFβ in the presence or absence of the PKCζ P.S or TAPI-2, as indicated. Endogenous C-terminal TβRI was visualized by immunofluorescence using the V22 antibody (TRITC). Quantification of the number of cells showing endogenous TβRI in the nucleus is shown on the right side of the panel (mean±s.d., n =3 independent experiment, where N=200-300 cells where counted in each group, * P <0.0003, ANOVA). Scale bar 20 μm. ( d ) Invasion assay for A549 cells treated with TGFβ in the absence or presence of TAPI-2 and PKCζ P.S. Cells were visualized by staining with crystal violet cell stain solution. Right panel presents mean values for OD of invasive cells. Error bars represents mean±s.d. ( n =3 independent experiments; * P <0.05, ** P <0.002, ANOVA). Full size image Nuclear TβRI ICD is observed in human tumours in vivo To explore whether nuclear accumulation of the TβRI ICD occurs in human tumours, we used immunohistochemistry to investigate the expression and localization of TβRI in a panel of prostate cancers, renal cell carcinomas and bladder tumours. Nuclear accumulation of TβRI ICD was observed in 19 of 19 investigated prostate cancer tissues, in 19 of 24 renal cell carcinomas, and in 21 of 23 bladder tumours, while staining with the H100 antibody to visualize the extracellular part of TβRI, showed staining only in the cytoplasm ( Fig. 8 ). No immunohistochemical staining of TβRI was observed in control experiment (when the primary antibodies were omitted, Supplementary Fig. S6 ). Thus, our data demonstrated that nuclear accumulation of TβRI ICD is observed in human tumours. 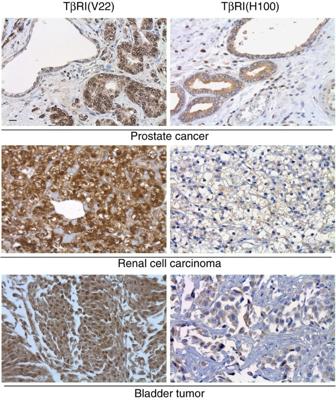Figure 8: TβRI ICD is localized in nucleus in different kinds of malignant tumours. Tumour tissues from prostate cancer, renal cell carcinoma and bladder tumour were stained with V22 and H100 antibodies, which recognize the intracellular and extracellular domain of TβRI, respectively. Scale bar 20 μm. Figure 8: TβRI ICD is localized in nucleus in different kinds of malignant tumours. Tumour tissues from prostate cancer, renal cell carcinoma and bladder tumour were stained with V22 and H100 antibodies, which recognize the intracellular and extracellular domain of TβRI, respectively. Scale bar 20 μm. Full size image We have provided evidence that TβRI undergoes cleavage by TACE in cancer cells and that the ICD of TβRI is translocated to the nucleus where it associates with the transcriptional regulator p300 in nuclear PML bodies. Accumulation of the ICD of TβRI in the nucleus occurs after TGFβ stimulation and is dependent on TRAF6, TACE and PKCζ. The expression levels of Smads did not influence the PKCζ-dependent generation of the ICD of TβRI as knock down of Smad4 by siRNA, had no effect on the PKCζ-induced generation of TβRI ICD ( Supplementary Fig. S7a ). Neither did overexpression of Smad2, 3 or 4 in PC-3U cells affect PKCζ-induced generation of TβRI ICD ( Supplementary Fig. S7b ). Since the TRAF6-binding deficient TβRI mutant (HA-E161A) still activates Smad2, while generation of the TβRI ICD is impaired, it appears that the canonical Smad pathway can operate independently of the generation of the TβRI ICD, which instead correlates with activation of the TRAF6—TAK1—p38 MAPK pathway ( Fig. 2a ). Integrins are essential adhesion receptors which are involved in cell migration and extracelullar matrix assembly [19] . TGFβ-induced activation of the p38 MAPK pathway has been demonstrated to be related to integrin signaling and implicated in epithelial-mesenchymal transition in certain cell lines [20] . To investigate a possible relationship between integrin signaling and TGFβ-induced generation of TβRI ICD, we used antibodies which promotes or inhibits integrin activation [21] (TS2 and CD29 antibodies, respectively). No major effects on TGFβ-induced formation of the TβRI ICD was observed, when integrins were activated or inhibited ( Supplementary Fig. S8 ). Exactly how TβRI ICD is translocated to the nucleus is the topic of our ongoing investigations. Interestingly, our finding that the ICD of TβRI associates with p300 and the Snail promoter, to support transcriptional regulation of a subset of genes, including Snail , MMP2 and p300 , correlates with increased invasiveness of cells. Whether the Smad proteins also participitate in the transcriptional complexes is an interesting possibility that remains to be elucidated. Nuclear accumulation of TβRI was observed in prostate, breast and lung cancer cells and also in several cancer tissues, but not in primary prostate epithelial cells. Thus the pathway elucidated in this report occurs in different kinds of human tumours and could contribute to tumour progression. Taken together, our data support the notion that the cleavage and nuclear accumulation of TβRI is part of a tumour promoting TGFβ signaling pathway. Cell culture The human prostate cancer cell lines PC-3U, originating from PC-3 [22] , which are known to produce TGFβ in an autocrine fashion [23] and LNCaP, were purchased from ATCC and grown in RPMI-1640 with 10% fetal bovine serum (FBS) and L-glutamine. Wt MEF and TRAF6 −/− MEF were grown in Dulbecco's modified Eagle's medium (DMEM) containing 10% FBS. Normal human primary prostate epithelial cells (PrEC) were purchased from Cambrex Bio Science Walkersville. The cells were grown according to the manufacturer's recommendation in Prostate Epithelial Cell Basal Medium supplemented with Clonetics PrEGM bullet kit. The cells were starved 12–18 h in medium supplemented with 1% FBS before TGFβ stimulation (TGFβ1 10 ng/ml (R&D System, UK). Antibodies and reagents Antibodies or antisera against the following proteins were used in immunoblotting or immunofluorescence (IF): HA (Y-11, 1:500 and 1:50 for IF), ubiquitin (P4D1, 1:400), TβRI (V22, 1:250 and 1:50 for IF); the specificity of this antibody has previously been reported [24] , [25] ) and H100 (1:250), TRAF6 (D10, 1:500) and p300 (NM11, 1:200) antibodies were from Santa Cruz Biotechonology; p-Smad2 (1:500) and TβRI (VPN, 1:500) antisera were generated in rabbits in-house; lamin A (1:1,000), TACE/ADAM17 (1:50 for IF), pPKCζ/λ (Thr410/403, 1:1,000), PKCζ (1:1,000), p-p38 (1:1,000), p38 (1:1,000), Smad2 (1:1,000) and acetyl-Lys antibodies (1:1,000) were from Cell Signaling. Antibody against TRAF6 C-term was from ZYMED Laboratories (1:500); UbK63 antibody (1:1,000) was from Enzo Life Sciences. UbK48 Clone Apu 207 antibody (1:1,000) was a kind gift from V.M. Dixit, Genetech; antibodies against β-actin (1:10,000), β-tubulin (1:1,000), HA (1:1,000) were from Sigma. The mouse monoclonal TS2/16 antibody (a kind gift from Dr K. Rubin) was used at a concentration of 20 μg/ml to activate β1-integrin and a rat anti-human CD29 antiserum, purchased from BD Pharmingen, was used at a concentration of 10 μg/ml to inactivate β1-integrin respectively. Horseradish peroxidase-coupled secondary antibodies were from Sigma. In some experiments, either goat anti-mouse IgG, light chain specific or mouse anti-rabbit IgG, light chain specific antisera from Jackson ImmunoResearch Laboratories, were used. 4,6-Diamidino-2-phenylindole dihydrochloride (DAPI) fluorescent dye to visualize cell nuclei by microscopy was purchased from Merck and TRITC labelled phalloidin from Sigma. Alexafluor 555 was purchased from Invitrogen. Protein-G Sepharose was from GE Healthcare; LumiLight Western blotting substrate and Pefabloc were from Roche, PageRuler prestained protein ladder was from Fermentas; TAPI-2 was from BIOMOL Research Laboratories Inc., and used at concentrations of 10–20 μM. PKCζ pseudosubstrate was from TOCRIS Bioscience. The PKC activator phorbol 12-myristate 13-acetate (PMA, referred to as TPA in our paper) and a TβRI inhibitor (SB505124), were purchased from Sigma and used at concentrations of 100 nM and 10 μM, respectively. All inhibitors were added 1 h before TGFβ stimulation. Protein analyses The cells were starved for 12–18 h and then stimulated with TGFβ for indicated time periods, washed twice in ice-cold PBS and lysed in ice-cold lysis buffer (150 mM NaCl, 50 mM Tris pH 8.0, 0.5% (v/v) DOC, 1% (v/v) NP40, 10% (v/v) glycerol, 1 mM aprotinin, 1 mM Pefabloc and 2 mM sodium orthovanadate). After centrifugation, supernatants were collected and protein concentrations were determined by BCA protein measurement kit (Nordic Biolabs). Equal amount of protein from total cell lysate and immunoprecipitation were run in SDS-PAGE using 6, 10, 12 or 4–12% gradient polyacrylamide gels, blotted on to polyvinylidine difluoride membranes and subjected to immunoblotting, as previously described [25] . In vitro and in vivo ubiquitination assays, immunofluorescence and transient transfections were performed, as previously described [5] , [26] , [27] . HA, TACE, H100 and V22 antibodies were diluted 1:50 when used for immunofluorescence. Photo micrographs were obtained by Zeiss 510 Meta (Carl Zeiss Microimaging, Inc.) with a digital camera (RET-EXi-F-M-12-C) from Q-imaging. Nuclear fractionation assays Two different protocols for nuclear fractionation were used to examine TβRI accumulation in the nucleus in response to TGFβ. The first used for cell fractionation, has earlier been described [27] and was used in the experiments shown in Figures 1b and 5d . The second was applied in experiments shown in Figure 3b and used Nuclear Complex Co-IP kit purchased from Active Motif. Cells in a 10-cm dish were washed twice with ice-cold PBS, and then scraped and collected into 1 ml ice-cold PBS; after centrifugation at 1,500 r.p.m. for 5 min at 4 °C, the cell pellet was gently resuspended in 500 μl Hypotonic Buffer and incubated on ice for 15 min. Twenty five μl of Detergent Solution was added and gently mixed and centrifuged at 14,000× g for 30 s, at 4 °C. The nuclear pellet was resuspended in 100 μl Complete Digestion Buffer, vortexed gently for 2 s after adding 0.5 μl of Enzymatic Shearing Cocktail, thereafter incubated for 10 min at 37 °C. The nuclear lysates were vortexed gently after 2 μl of 0.5 M EDTA had been added to stop the reaction, and then incubated on ice for 5 min, centrifuged (14,000 g , 10 min, 4 °C), and the supernatant was collected for immunoprecipitation. Invasion assay Invasion assays were performed by using the CytoSelect™ Cell Invasion Assay (Cell Biolabs, Inc., San Diego, CA). The basement membrane layer of the cell culture inserts were rehydrated in 300 μl serum-free RPMI-1640, and 2×10 6 cells were seeded into the upper area of the chambers in serum-free RPMI-1640 with or without TGFβ. Lower wells of the invasion plates were filled with 500 μl RPMI, supplemented with 10% FBS. Non-invasive cells were removed from the upper chamber and invasive cells were photographed by a Leica DMR light microscope, after staining with crystal violet cell stain solution. Colorimetric quantification was performed by transfer inserts into 200 μl of extraction solution for 10 min. Optical density (O.D.) at 560 nm was determined for extracts transferred to a 96-well microtiter plate using a plate reader. Plasmids and DNA transfections GFP-caTβRI was constructed by cloning full length caTβRI between the immediate early promoter of CMV and the EGFP coding sequence; the C-terminus of caTβRI was fused to the N-terminus of pEGFP-N3 vector. The pcDNA3 and wt PKCζ plasmids were from Addgene. HA-caTβRI and HA-TβRI KR (kinase dead (KD) mutant) with HA fused to the C-terminus of TβRI, were kind gifts from P. ten Dijke (University of Leiden, The Netherlands). Expression vectors for C-terminally tagged HA-tagged G120I mutant for caTβRI were generated by PCR and the mutation was confirmed by sequencing. The caTβRI-E161A plasmid with HA fused to the C-terminus of TβRI was described before [5] . HA-TβRI with HA inserted between amino acid residues 27 and 28, was a kind gift from Dr S. Corvera (University of Massachusetts Medical School, Worcester, USA). 3xHA-tagged wild-type ubiquitin, K48- and K63-only ubiquitin mutants were kind gifts from V.M Dixit (Genentech, San Francisco, CA). Expression vector for GST-TβRI fusion protein, encoding the complete cytoplasmic part (amino acid 148-503) of ca TβRI (T204D) has been described previously [28] . siRNA transfection Twenty-one-base pair siRNA duplexes for TβRI (also known as ALK5), SMART pool siRNA for TRAF6 as previously described [5] , and a non-specific control siRNA, were synthesized by Dharmacon Research (Lafayette, CO). The sequence for TβRI siRNA duplex was 5′ AAC AUA UUG CUG CAA CCA GGA 3′, and the non-specific duplex oligo 5′ AAC AGU CGC GUU UGC GAC UGG 3′. PKCζ siRNA (h2) was from Santa Cruz biotechnology. The siRNA was transfected with Oligofectamine (Invitrogen) according to the manufacturer's protocol. Expression analysis Total RNA was isolated from cells using RNeasy Minikit (Qiagen) and Thermoscript RT–PCR System (Invitrogen) was used for the preparation of double-stranded cDNA. qRT–PCR was performed using Power SYBR Green PCR Mastermix (Applied Biosystems) with the Stratagene MX3000P. The following primers were used for qRT–PCR. TβRI, forward primer (FP), TGTTGGTACCCAAGGAAAGC, reverse primer (RP), CACTCTGTGGTTTGGAGCAA; p300, FP, GGGACTAACCAATGGTGGTG, RP, GTCATTGGGCTTTTGACCAT; SNAIL 1, FP, GAGCATACAGCCCCATCACT, RP, GGGTCTGAAAGCTTGGACTG; Smad7, FP, TCCTGCTGTGCAAAGTGTTC, RP, TCTGGACAGTCTGCAGTTGG; MMP 2, FP, AGGCCGACATCATGGTACTC, RP, GGTCAGTGCTGGAGAAGGTC; PAI 1, FP,CTCTCTCTGCCCTCACCAAC, RP, GTGGAGAGGCTCTTGGTCTG. Chromatin immunoprecipitation ChIPs were performed for three or more biological replicates. The ChIP protocol provided by Abcam, Cambridge UK was followed. The chromatin was precipitated using the V22 rabbit antibody (Santa Cruz). After purification, the DNA was amplified using qRT-PCR to analyze ChIP DNA in triplicate. The following primers were used for ChIP; Snail1 forward primer, GGACTCAGGGAGACTCATGG, reverse primer, GGGTCTACGGAAACCTCTGG. Histology of human tumours Tissue microarrays (TMAs) of malignant tissues, containing multiple samples from different patients with prostate cancer, renal cell carcinoma and bladder cancer produced by the Human Proteome Atlas (HPA) facility ( http://www.proteinatlas.org ) were stained using anti-TβRI antibodies (V22 and H100). Pictures of stained TMA sections were taken with an ALTRA 20 soft imaging system and an Olympus BX45 microscope. Ethical permit to use decoded, tumour tissues for generation of tissue slides or TMA was granted by the Uppsala ethical review board in full agreement with the Swedish Ethical Review Act. Statistical analysis P values were calculated by Student's two-tailed t -test or One-way ANOVA, as indicated in Figure legends. Analyses were performed in a Statistica software program. Values are expressed as mean±s.d., of three or more independent experiments performed in triplicates, unless otherwise indicated. P values of <0.05 were considered statistically significant. How to cite this article: Mu, Y. et al . TRAF6 ubiquitinates TGFβ type I receptor to promote its cleavage and nuclear translocation in cancer. Nat. Commun. 2:330 doi: 10.1038/ncomms1332 (2011).